Power-controlled transition from standard to negative refraction in reorientational soft matter Refraction at a dielectric interface can take an anomalous character in anisotropic crystals, when light is negatively refracted with incident and refracted beams emerging on the same side of the interface normal. In soft matter subject to reorientation, such as nematic liquid crystals, the nonlinear interaction with light allows tuning of the optical properties. We demonstrate that in such material a beam of light can experience either positive or negative refraction depending on input power, as it can alter the spatial distribution of the optic axis and, in turn, the direction of the energy flow when traveling across an interface. Moreover, the nonlinear optical response yields beam self-focusing and spatial localization into a self-confined solitary wave through the formation of a graded-index waveguide, linking the refractive transition to power-driven readdressing of copolarized guided-wave signals, with a number of output ports not limited by diffraction. Light refraction at dielectric interfaces under the Snell–Descartes law is among the best known concepts in optics, its theoretical basis stemming from Maxwell’s equations and momentum conservation [1] . Ray-tracing techniques and the design of several optical devices rely on refraction. In isotropic media and at frequencies well removed from absorption regions, incident and refracted rays at an interface always lie on opposite sides of the normal to it, that is, they undergo standard (positive) refraction or, simply, refraction. Some natural and man-made media can also exhibit negative refraction, when both impinging and refracted rays belong to the same half-plane [2] . Owing to the conservation of momentum across the interface, negative refraction requires a nonzero walk-off angle between the phase velocity v p and the group velocity v g in the medium hosting the refracted beam. Two main types of light–matter interactions can satisfy this requirement: with backward waves when v p · v g ≪ 0, or with forward waves when v p · v g >0, respectively [2] . The case of backward waves corresponds to the so-called negative refractive index, a counterintuitive phenomenon occurring in absorptive media or in metamaterials [3] , [4] . In the first decade of the twentieth century, Schuster (following W. Lamb’s original idea in mechanical systems) studied negative refraction considering backward waves in the presence of a lossy medium at an interface, and predicted its unobservability due to the evanescent character of the involved waves [5] . Nearly one century later, negative refraction was revived by Pendry’s seminal paper on the superlens effect based on amplified evanescent waves in a metamaterial [6] . Negative refraction in metamaterials has been recently demonstrated at microwave [7] , [8] as well as near-infrared [9] , visible [10] and ultraviolet wavelengths [11] . Surfing this wake of interest, researchers have also investigated negative refraction with forward waves, devoting special attention to photonic crystals [12] , [13] and natural anisotropic media [14] , [15] . In the latter class of materials, where double refraction was first described by E. Bartholinus in the seventeenth century [16] , negative refraction stems from birefringent walk-off when the Poynting vector (directed as the energy flux) lies on the opposite side of the refracted wavevector with respect to the normal at the interface [2] . The superlens effect in natural non-absorbing crystals is ruled out by the cutoff on transverse wavevectors (it might survive in photonic crystals when photons have a negative effective mass [12] and behave as in a hyperbolic material [17] ); nonetheless, negative (or backward) refraction remains relevant as it can maximize the angular beam deflection associated with impedance matching at an interface [14] . In this scenario, anisotropic soft matter—such as liquid crystals—has been used in the pursuit of electrically-adjustable negative refraction with either diffracting [18] , [19] or self-confined beams [20] . In this article, we report on nonlinear refraction with forward wavepackets in uniaxial nematic liquid crystals (NLCs): we obtained standard and negative light refraction at an interface using a single extraordinary polarization and were able to nonlinearly control the transition from one (positive) to the other (negative) by exploiting the walk-off dependence on beam power. At variance with previous attempts based on wave mixing [15] , [21] , in NLCs the optic axis can undergo reorientation by light self-action with continuous-waves at mW powers, achieving self-tunability of the beam direction, that is, self-steering: as the incident power increases, nonlinear walk-off modifies the light path and steers the refracted beam to the opposite side of the interface normal, achieving negative refraction with overall angular deflections as large as 7°. Moreover, reorientation is accompanied by self-focusing with beam self-localization into spatial solitary waves [22] : these are self-induced waveguides that permit to balance out the diffractive spreading, enhance the all-optical response, guide copolarized signals of different wavelengths and maximize the transverse resolution on steering, that is, the number of resolvable output spots or signal exit ports. Self-steering and negative refraction in NLCs NLCs are states of matter sharing the properties of both solid-state crystals and liquids: they exhibit orientational order with the constituent elongated molecules randomly distributed in position [23] . The molecular orientation is macroscopically described by a space/time-dependent vector field, the molecular director , collinear with the average alignment of the main (long) molecular axes. At optical frequencies, most NLCs are positive uniaxials with their optic axis along , extraordinary refractive index for electric fields oscillating parallel to and ordinary index for fields normal to , respectively. NLCs exhibit a giant all-optical response observable with low-power continuous-wave excitations [24] , the reorientational optical nonlinearity: a suitably (extraordinarily) polarized electric field can induce molecular dipoles and make them reorient within the principal plane in order to minimize the system energy in the presence of elastic (intermolecular) interactions [23] , [24] . Such reorientational response is at the basis of a number of observed phenomena, ranging from bistability [25] to pattern formation [26] , generation of complex topological structures [27] , [28] , [29] or light-controlling-light; in particular, the latter has been exploited—at mW and sub-mW power levels—for generating, controlling and routing ‘nematicons’, that is, spatially self-localized beams stemming from the balance between transverse spatial dispersion (diffraction) and self-focusing [22] . NLCs are ideal candidates for the observation of nonlinear negative refraction: they are highly birefringent (typically in the visible spectrum), with walk-off (angular departure of Poynting vector from wavevector) as large as ≈7°, thus enhancing the role of anisotropy at dielectric interfaces [30] , [31] ; moreover, they are transparent from infrared to ultraviolet, with losses mainly due to Rayleigh scattering [23] , [24] ; finally, their response is such that a non-perturbative nonlinear regime can be experimentally accessed in the context of classical optics [32] . The basic configuration for studying nonlinear tunable refraction from standard to negative in NLCs is sketched in Fig. 1 . A thick NLC layer is homogeneously aligned in a planar cell with director along the axis z normal to the input interface in z =0. A light beam is launched across the air-(glass)-NLC interface with input wavevector k in at an angle β in with respect to z ; its electric field E oscillates in the principal plane yz of the uniaxial NLC and excites extraordinary waves. The system has mirror symmetry with respect to z , thus the light evolution is unaffected by the transformation β in → − β in . Fig. 1 illustrates the case β in ≪ 0: the Snell–Descartes law provides the implicit equation β =arcsin [sin β in / n e (− β )] for the refraction angle β , where depends on the angle θ between and k ; in the linear regime θ corresponds to − β . 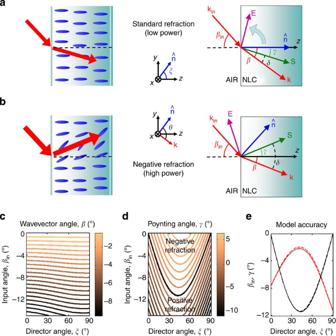Figure 1: Basic configuration and initial assessment of the phenomenon. An extraordinarily polarized light beam impinges on the air-(glass)-NLC interface defining the input to the planar cell. (a) At low powers, the molecular director is parallel tozand positive refraction occurs for any incidence angleβinof wavevectorkin. (b) As the input beam power increases, the reorientational torque rotates the directortowards theE-field vector (as indicated by the curved arrow ina), reducing the angle of refraction |β| and increasing the walk-offδ, eventually resulting in negative refraction when |βin| gets small enough. All angles are defined positive when taken clockwise with respect to thexaxis:βremains negative regardless of the type of refraction, whereasγchanges sign in the transition from positive (Poynting vectorSin they≪0 half-plane) to negative (Sin they>0 half-plane) refraction. Insets: definitions of (lower inset) angleθbetweenkand(positive in the example) and (upper inset) angleξbetweenandz. (c) Contour plot of wavevector angleβand (d) contour plot of Poynting vector angleγversus director orientationξand incidence angleβin; the black solid line in (d) corresponds to a Poynting vector alongz(that is,γ=0). (e) Graph of the largestβinversusξ(black lines) corresponding toγ=0 (that is, maximum angle of incidence to support negative refraction, black line ind) andγversusξforβin=−15° (red lines), respectively; solid and dashed lines are exact and approximate solutions, respectively. Here=1.7 and=1.5; the wavelength of light isλ=1.064 μm. Figure 1: Basic configuration and initial assessment of the phenomenon. An extraordinarily polarized light beam impinges on the air-(glass)-NLC interface defining the input to the planar cell. ( a ) At low powers, the molecular director is parallel to z and positive refraction occurs for any incidence angle β in of wavevector k in . ( b ) As the input beam power increases, the reorientational torque rotates the director towards the E -field vector (as indicated by the curved arrow in a ), reducing the angle of refraction | β | and increasing the walk-off δ , eventually resulting in negative refraction when | β in | gets small enough. All angles are defined positive when taken clockwise with respect to the x axis: β remains negative regardless of the type of refraction, whereas γ changes sign in the transition from positive (Poynting vector S in the y ≪ 0 half-plane) to negative ( S in the y >0 half-plane) refraction. Insets: definitions of (lower inset) angle θ between k and (positive in the example) and (upper inset) angle ξ between and z . ( c ) Contour plot of wavevector angle β and ( d ) contour plot of Poynting vector angle γ versus director orientation ξ and incidence angle β in ; the black solid line in ( d ) corresponds to a Poynting vector along z (that is, γ =0). ( e ) Graph of the largest β in versus ξ (black lines) corresponding to γ =0 (that is, maximum angle of incidence to support negative refraction, black line in d ) and γ versus ξ for β in =−15° (red lines), respectively; solid and dashed lines are exact and approximate solutions, respectively. Here =1.7 and =1.5; the wavelength of light is λ =1.064 μm. Full size image Common NLCs are positive uniaxials with Δ n >0; hence, the Poynting vector is always coplanar with the wavevector k and the optic axis , and lies between them. The walk-off angle is , with the optical anisotropy; therefore, δ and θ have the same sign. Defining γ the angle of the Poynting vector with z , in the linear regime it is γβ >0, that is, light rays undergo positive refraction for every incidence angle β in . In the nonlinear regime, conversely, the reorientation of the optic axis can affect the beam (ray) direction. With reference to Fig. 1 , an extraordinarily polarized light beam can induce a rotation of the molecular director away from the wavevector, in turn increasing the size of the walk-off | δ |. Even if β remains negative for every angle ξ between and z , since θ = ξ−β the Poynting vector can change side with respect to z , giving rise to negative refraction when | δ |>| β |. From Fig. 1 and the Snell–Descartes law, it is straightforward to obtain the refraction angle for light rays as In the limit of small incidence angles β in , equation (1) gives where we set . Neglecting the terms containing powers of ε a larger than 2, it stems from equation (2) that negative refraction can only occur if Figure 1c,d graph wavevector and Poynting vector angular directions in the NLC versus the two free parameters, that is, director orientation ξ and angle of incidence β in (in the interval [−15° 0°]); we set =1.7 and =1.5 as in the E7 mixture at 1064, nm (ref. 33 ). When | β in | ≪ 5°, the refraction angle β slightly changes with ξ , never exceeding variations of 1°; negative refraction occurs for small β in , with smaller β in corresponding to larger negative refraction. Figure 1e compares approximate (from equation (2)) and exact solutions (from equation (1)) for γ in the (worst) case β in =−15°; in the same figure (red lines) the validity of equation (3) is apparent in calculating the maximum input beam tilt, which permits the observation of negative refraction. Exact and approximate results are mutually consistent to a good accuracy. Experimental verification To validate our prediction with experiments, we prepared a planar glass cell of thickness L =100 μm across x , filled it with the E7 mixture (Δ n ≈0.2) and sealed the input to ensure a homogeneous director distribution and the absence of a meniscus [22] . The molecular director was aligned along the normal z to the input interface, as in Fig. 1a . Due to the cell shape, the sample was subject to one-dimensional boundary effects versus x but could be considered infinitely extended across y (ref. 34 ). A TEM 00 laser beam of wavelength λ =1.064 μm was gently focused into the sample, slightly past the input glass/NLC interface to avoid spurious interactions with the molecules anchored at the boundary; the input waist was set to w 0 ≈8 μm by using two lenses in a telescopic arrangement and a microscope objective. Two mirrors (M 1 and M 2 in Fig. 2 ) ensured accurate control of the input conditions, particularly the incidence angle β in . 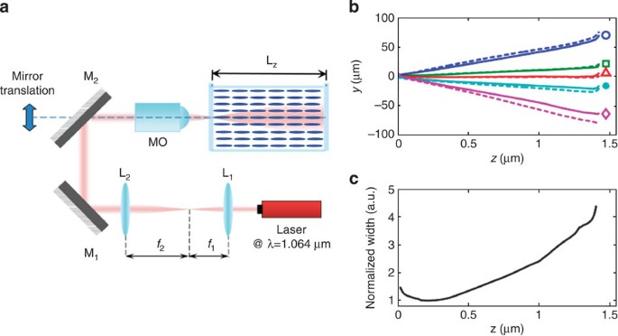Figure 2: Setup and linear characterization. (a) Sketch of the experimental set-up: lenses L1and L2form a telescope; mirror M1is fixed, mirror M2can be translated to adjust the beam path and the incidence angle. (b) Beam trajectories in the linear limit (2 mW input power) forβin=0° (red line with triangle), ±1.5° (green line with square and cyan line with star) and ±5° (blue line with circle and magenta line with diamond); solid and dashed lines correspond to extraordinary and ordinary waves, respectively. (c) Normalized beam widthw/w0versuszat normal incidence forβin=0° and 2 mW input power. Herew0=8 μm. Figure 2: Setup and linear characterization. ( a ) Sketch of the experimental set-up: lenses L 1 and L 2 form a telescope; mirror M 1 is fixed, mirror M 2 can be translated to adjust the beam path and the incidence angle. ( b ) Beam trajectories in the linear limit (2 mW input power) for β in =0° (red line with triangle), ±1.5° (green line with square and cyan line with star) and ±5° (blue line with circle and magenta line with diamond); solid and dashed lines correspond to extraordinary and ordinary waves, respectively. ( c ) Normalized beam width w / w 0 versus z at normal incidence for β in =0° and 2 mW input power. Here w 0 =8 μm. Full size image The beam-to-cell alignment was monitored by acquiring the trajectories of extraordinary and ordinary rays propagating in the linear regime ( Fig. 2b ), using a CCD (charge-coupled device) camera to collect the out-of-plane ( yz ) scattered light; the acquired beam paths could then be compared with the calculated ones ( Fig. 1c,d ; ref. 35 ). A second CCD camera was used to acquire the output profile through the exit facet of the sample. Fig. 2c shows the measured beam width, defined as , versus z in the linear regime and normalized with respect to w 0 ; A is the amplitude of the light wavepacket. In the described conditions (cell configuration, beam waist, small β in and low power), beam propagation was ruled by diffraction, with a Rayleigh distance of ≈280 μm. When the optical excitation is larger (in the highly nonlinear regime), nonlinear refraction can take place: the director orientation ξ depends on the input power through optical reorientation, providing in turn a change in walk-off [36] ; in addition, a (smaller) nonlinear correction of β is caused by the increase of the extraordinary refractive index n e ( β ) (see Eq. (1) and Fig. 1c ). Therefore, for high-enough excitations the light beam can adjust the direction of its own Poynting vector by altering the walk-off. 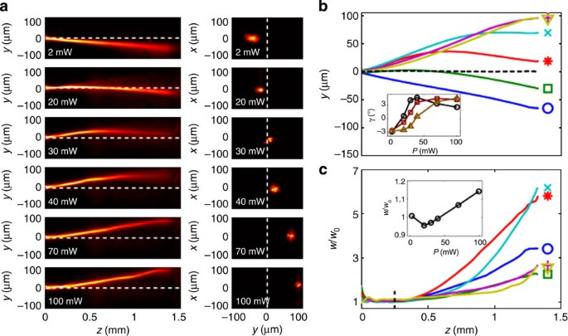Figure 3: Demonstration of nonlinear negative refraction. (a) Beam evolution in the observation planeyz(left) and output profiles in the transverse planexy(right) whenβin=−4.9°. The dashed line indicates the cell mid-sectiony=0. (b) Corresponding trajectories and (c) normalized beam width versuszfor an input power of 2 mW (blue line with circle), 20 mW (green line with square), 30 mW (red line with star), 40 mW (cyan line with cross), 70 mW (magenta line with plus) and 100 mW (yellow line with inverted triangle). The black dashed line inbindicates the trajectory in the linear regime when |βin|≈0° within the experimental accuracy. Inset inb: angleγversus input power, measured inz=150 μm (black line with circle),z=500 μm (clay line with square) andz=1 mm (mustard line with triangle). Inset inc: normalized beam width versus power measured inz=250 μm. Figure 3a displays the acquired images of beam evolution and output profile for β in =−4.9°. As expected, the beam moves sideways versus input power. At variance with the predictions of equation (2), however, it does not propagate straight when steered by way of nonlinear walk-off: the observed bending is due to scattering losses, which cause a reduction in beam power versus z , hence a reduced nonlinear response with progressively vanishing reorientation [36] . In particular, for P ≈30 mW the beam positions at sample input and output nearly coincide, with an apparent γ =0 resulting at the exit. Further increases in input power allow for negative refraction, that is, the outgoing beam can be seen to emerge in the same half-plane y >0 of the incident beam (rightmost panels of Fig. 3a for P >30 mW). Figure 3: Demonstration of nonlinear negative refraction. ( a ) Beam evolution in the observation plane yz (left) and output profiles in the transverse plane xy (right) when β in =−4.9°. The dashed line indicates the cell mid-section y =0. ( b ) Corresponding trajectories and ( c ) normalized beam width versus z for an input power of 2 mW (blue line with circle), 20 mW (green line with square), 30 mW (red line with star), 40 mW (cyan line with cross), 70 mW (magenta line with plus) and 100 mW (yellow line with inverted triangle). The black dashed line in b indicates the trajectory in the linear regime when | β in |≈0° within the experimental accuracy. Inset in b : angle γ versus input power, measured in z =150 μm (black line with circle), z =500 μm (clay line with square) and z =1 mm (mustard line with triangle). Inset in c : normalized beam width versus power measured in z =250 μm. Full size image For a better assessment of the phenomenon, Fig. 3b,c plot the beam trajectories and normalized widths versus z , corresponding to Fig. 3a . The paths change non-monotonically with power due to the δ dependence on θ , with a maximum δ for θ ≈45° ( Fig. 1d ). The combined effect of (scattering) losses and nonlinear walk-off is responsible for the change (in both amplitude and sign) of the initial slope of the trajectories. As stated above, a stronger reorientation corresponds to a larger walk-off up to its maximum, with the opposite trend for further (nonlinear) increases in θ : the analysis of the trajectories ( Fig. 3b ) and their slope (inset Fig. 3b ) allows estimating an angle θ ≈45° near the input interface for powers slightly above P =40 mW. For P =30 mW the angle γ results positive up to z ≈600 μm, then retrieves its linear value owing to vanishing reorientation, as losses reduce the local beam power. For P ≈40 mW the maximum orientation is≈45°: γ monotonically decreases along z , going from positive to negative values after a propagation distance z which lengthens with power. For P >70 mW the initial γ reduces as power increases, conserving its sign along z . Eventually, for P ≈100 mW, the Poynting vector angle γ monotonically increases versus z up to a maximum, with θ ≈45° at the output. Furthermore, the measured beam width confirms the occurrence of light self-trapping, more and more effective as power increases ( Fig. 3c ). For P =30 mW and P =40 mW, when the beam profile gets narrower (that is, self-confinement is stronger, inset in Fig. 3c ), the outgoing beam results wider due to the stronger diffraction after losses prevail on self-focusing. In particular, the minimum waist is obtained for P =40 mW, confirming the value of θ ≈45° inferred from Fig. 3b when the nonlinearity is maximized. For P =100 mW, in the early stages of propagation the beam is wider than at lower powers due to saturation of the nonlinear response ( θ >45° (ref. 32 )). The power-controlled steering action is shown in Fig. 4 , for the case β in =−4.9°. Clearly, in the solitary regime the beam size is of the order of the input width (see inset), permitting to resolve a large number of output positions versus y , that is, a number of output ports for signals guided by solitons. Careful engineering (reducing input waist and scattering losses, increasing wavelength and propagation distance) could easily result in spatial readdressing to >30 output channels with negligible crosstalk. 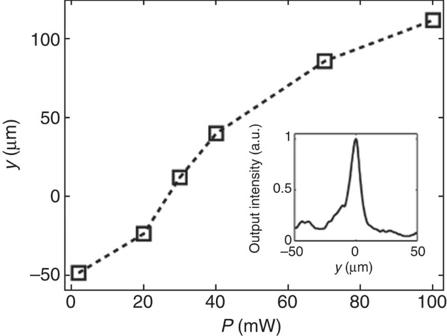Figure 4: Power-dependent beam refraction and steering. Output beam position on theyaxis versus input power, for an angle of incidenceβin=−4.9°. The self-confined beam and the associated graded-index waveguide undergo angular steering and transverse displacement versus excitation. The resulting power-controlled router has a number of output ports (and outgoing guided-wave signals) defined by the overall angular span and the width of the self-trapped beam. The inset shows a typical self-guided (solitary) beam profile (P=30 mW). Figure 4: Power-dependent beam refraction and steering. Output beam position on the y axis versus input power, for an angle of incidence β in =−4.9°. The self-confined beam and the associated graded-index waveguide undergo angular steering and transverse displacement versus excitation. The resulting power-controlled router has a number of output ports (and outgoing guided-wave signals) defined by the overall angular span and the width of the self-trapped beam. The inset shows a typical self-guided (solitary) beam profile ( P =30 mW). Full size image The experimental results on nonlinear beam refraction are summarized in Fig. 5 : the output beam position in y changes with input power for various incidence angles β in . Nonlinear negative refraction is largest for small β in , consistently with Fig. 1d . The maximum nonlinear deflection of the beam was obtained for a finite β in , rather than the predicted β in =0, because powers above an upper value caused the beam to wiggle strongly due to temporal instabilities in the medium [37] , [38] . 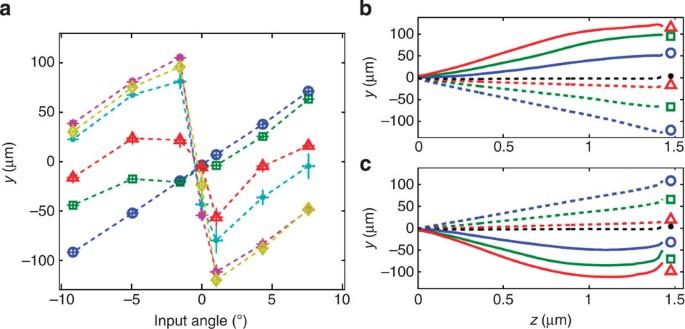Figure 5: Nonlinear refraction and its mirror symmetry versus incidence angle. (a) Output beam position inyversusβin, measured inz=1.1 mm for an input power of 2 mW (blue with circle), 20 mW (green with square), 30 mW (red with triangle), 40 mW (cyan with dot), 70 mW (magenta with star) and 100 mW (yellow with diamond). (b) Beam paths forβin≪0 and (c) beam paths forβin>0: input powers are 2 mW (linear case, dashed lines) and 70 mW (solitary wave propagation, solid lines). The incidence angles forβin≪0 (βin>0) are −9.2° (7.6°) (blue with circle), −4.9° (4.3°) (green with square), −1.6° (1.0°) (red with triangle). The dashed black lines with dot are the paths corresponding toβin≈0°. Figure 5a is not perfectly symmetric due to the unavoidable sample imperfections and the finite experimental accuracy. For an input power of 100 mW, the graph shows a maximum nonlinear deflection of about 150 μm, the largest self-steering obtained to date (significantly larger than in ref. 36 ) via power-dependent walk-off. Finally, we checked the mirror symmetry of our sample by comparing the experimental data for positive and negative β in : the plots in Fig. 5b,c confirm that, within measurement errors, the system is specularly symmetric. Figure 5: Nonlinear refraction and its mirror symmetry versus incidence angle. ( a ) Output beam position in y versus β in , measured in z =1.1 mm for an input power of 2 mW (blue with circle), 20 mW (green with square), 30 mW (red with triangle), 40 mW (cyan with dot), 70 mW (magenta with star) and 100 mW (yellow with diamond). ( b ) Beam paths for β in ≪ 0 and ( c ) beam paths for β in >0: input powers are 2 mW (linear case, dashed lines) and 70 mW (solitary wave propagation, solid lines). The incidence angles for β in ≪ 0 ( β in >0) are −9.2° (7.6°) (blue with circle), −4.9° (4.3°) (green with square), −1.6° (1.0°) (red with triangle). The dashed black lines with dot are the paths corresponding to β in ≈0°. Full size image We reported on the first experimental observation of nonlinear refraction—from positive to negative — by beam self-action in reorientational NLCs, supported by walk-off dependence on beam power when the nonlinear response becomes comparable with the linear one. While both light self-deflection and nonlinear negative refraction could be observed in other anisotropic media with a reorientational nonlinearity [39] , our geometry in NLCs optimizes their observation and characterization in highly nonlinear and highly anisotropic soft matter. This work may impact in the study of light-matter interactions towards the design and realization of novel light-controlling-light devices and systems. Here nonlinear refraction is obtained through self-confinement and solitary wave propagation at relatively low powers; hence, self-trapped optical wavepackets in space enhance the nonlinear response and make this configuration appealing towards power-steerable waveguides or reconfigurable interconnects, where the same optical element realizes both signal guidance and control. Accessing the negative refraction regime enables to maximize the total angular span of such waveguide steering, permitting to resolve a large number of output ports (channels) and increase the system capacity. As further developments, we envisage the generalization of the phenomena here shown to, for example, optomechanical meta-atoms [39] , [40] , soft matter with metallic nanoparticles [41] , solutions of graphene-oxide flakes [42] . We also foresee fascinating new phenomena stemming from the combined effects of artificial magnetoelectric coupling in metamaterials and natural dielectric anisotropy, for example, exploring the tunability of liquid crystals-based metamaterials [43] , where the interplay of nonlinear refraction (discussed hereby) and a negative refractive index or negative diffraction could be exploited towards novel exotic phenomena. Modeling light propagation in the nonlinear regime In the nonlinear regime, in the absence of losses and under the single elastic constant ( K ) approximation [24] , an extraordinarily polarized electromagnetic wave in the harmonic regime at pulsation ω propagates in reorientational uniaxial NLC according to where ε ij are Cartesian components of the dielectric tensor, μ 0 is the magnetic permeability of vacuum, H and E are the magnetic (linearly polarized along x ) and electric (polarized in yz ) fields, respectively; the subscript t in equation (6) refers to the local polarization of the electric field, in turn determined by γ . Owing to the highly nonlocal response of NLC [22] , [24] , all the dielectric parameters in equations (4, 5, 6) can be evaluated on the beam axis, except for , which is responsible of self-focusing [32] . Thus, the walk-off angle is δ ( ξ max − β ), with ξ max ( z ) the maximum reorientation at the field peak on each z . Sample preparation The planar cells used in the experiments consist of two parallel glass slides placed normal to the x axis, measuring 1.5 and 40 mm along z and y , respectively: the length along z allows observing the output profiles despite scattering losses; the width along y allows preventing boundary effects. The cell thickness across x , L x =100 μm determined by Mylar spacers, ensures both bulk-like beam propagation and operation in the highly nonlocal regime [32] . Both slides were covered by a polymer (polyvinyl carbazole doped with C60) thin film and mechanically rubbed along z in order to ensure the planar alignment of the molecular director along the z axis, with a pretilt angle ≈0°, as measured by the crystal rotation method [44] . The cell was uniformly filled with the commercial nematic mixture E7 by capillarity. To maximize the coupling of the input laser beam to the extraordinary wave component in the NLC layer, two additional glasses of thickness 100 μm were attached to the edges of the cell (perpendicular to z in z =0 and z =1.5 mm) using ultraviolet curable glue after depositing a thin polyimide layer; these two glasses were treated to induce homeotropic alignment, thus ensuring a homogeneous director distribution in absence of external stimuli. Such input and output glass facets prevented the formation of NLC menisca and undesired beam depolarization at the input, as well as degradation of the sample in time. Experimental set-up Accurate measurements of beam incidence were carried out by calibrating the angular deflection of the beam after the microscope objective (MO) against the lateral shift of the mirror (M 2 , Fig. 2a ), mechanically controlled with a resolution of 1 μm. The sample was placed as close as possible to MO in order to minimize changes in the impact point, the latter changes being detrimental when trying to avoid artifacts associated with possible inhomogeneities in director distribution at the input facet. The input beam direction corresponding to the optimum parallelism between the input wavevector and the z axis (normal to the input facet) was achieved by maximizing the overlap of the trajectories of ordinary (input polarization along x ) and extraordinary (input polarization along y ) components in the sample at low powers (linear regime): ordinary- and extraordinary-wave Poynting vectors are collinear when the initial wavevector is parallel to the optic axis. The evolution (plane yz ) and output profiles (plane xy ) of the beams were imaged by single-shot acquisitions of the out-of-plane scattered light and intensity distribution at the exit facet, respectively. The measured trajectories and beam widths were averaged over several acquisitions to reduce the impact of noise. How to cite this article: Piccardi, A. et al. Power-controlled transition from standard to negative refraction in reorientational soft matter. Nat. Commun. 5:5533 doi: 10.1038/ncomms6533 (2014).